Intermolecular diastereoselective annulation of azaarenes into fused N-heterocycles by Ru(II) reductive catalysis Derivatization of azaarenes can create molecules of biological importance, but reductive functionalization of weakly reactive azaarenes remains a challenge. Here the authors show a dearomative, diastereoselective annulation of azaarenes, via ruthenium(II) reductive catalysis, proceeding with excellent selectivity, mild conditions, and broad substrate and functional group compatibility. Mechanistic studies reveal that the products are formed via hydride transfer-initiated β -aminomethylation and α -arylation of the pyridyl core in the azaarenes, and that paraformaldehyde serves as both the C1-building block and reductant precursor, and the use of Mg(OMe) 2 base plays a critical role in determining the reaction chemo-selectivity by lowering the hydrogen transfer rate. The present work opens a door to further develop valuable reductive functionalization of unsaturated systems by taking profit of formaldehyde-endowed two functions. Azaarenes constitute a class of ubiquitously distributed substances applied in numerous fields of science and technology [1] , [2] . The development of new strategies enabling efficient and selective transformation of weakly reactive azaarenes into functional frameworks is of important significance, as they not only pave the avenues to access novel functional products, but also enrich the synthetic connotation of the azaarenes. To date, except the well-established electrophilic substitution utilizing azaarenes as the nucleophiles under harsh conditions [3] , [4] , the recently emerged C–H bond activation/functionalization has offered many desirable ways for structural modification of the azaarenes [5] , [6] , [7] . In comparison with these aromaticity-retaining transformations, only a handful examples focused on dearomative coupling of active indole derivatives [8] , [9] , [10] , [11] , whereas dearomative functionalization of inert pyridine-fused azaarenes (e.g., quinolines, isoquinolines, naphthyridines, phenanthroline, etc.) [12] , [13] , [14] has been scarcely explored. In recent years, hydrogen transfer-mediated coupling reactions have emerged as appealing tools in the production of various functional products, since there is no need for high pressurized H 2 and elaborate experimental setups. For instance, in addition to the well-known reductive amination applied for amine syntheses [15] , [16] , several groups such as Beller [17] , [18] , Kempe [19] , [20] , Kirchner [21] , [22] , Liu [23] , [24] , [25] , and others [26] , [27] , [28] , [29] have applied borrowing-hydrogen strategy to alkylate amines and the α -site of carbonyl compounds with alcohols. Krische has demonstrated elegant contributions on the linkage of alcohols/carbonyls with unsaturated C–C bonds [30] , [31] , [32] . Bruneau et al. have achieved β -C(sp 3 )−H alkylation of N-alkyl cyclic amines [33] , [34] . The Li group has converted phenols into synthetically useful amines [35] , [36] . Our group has reported a reductive quinolyl β -C–H alkylation with a low-active heterogeneous cobalt catalyst [37] . Later, Donohoe et al. have demonstrated interesting examples on the β -functionalization of azaarenes [38] , [39] , [40] . Despite these important advances, the strategy incorporating a tandem coupling sequence into the reduction of azaarenes remains to date a challenge due to the difficulty in controlling the reaction selectivity: on one hand, the azaarenes tend to undergo direct hydrogenation to form non-coupled cyclic amines under catalytic reduction conditions, on the other hand, it is hard to selectively transfer hydrogen only to one specific sites among different substrates. Here, we conceived that, through an initial N-alkylation of azaarenes A′ with bromoalkanes to form azaarenium salts [41] , [42] , a solution to achieve the desired synthetic purpose would be offered: (i) the combination of a suitable metal catalyst (M) and hydrogen donor (HD) forms reductive metal hydride species [HM n X] in-situ, which allows hydride transfer (TH) to the azaarenium salts A to generate allylic amine int-1 and its tautomer N-alkyl enamine int-2 (Fig. 1a ). Such an enamine ( int-2 ) has higher β -reactivity in trapping electrophiles than its −NH counterpart and lowers the formation of non-coupled cyclic amine A ″. (ii) It is relatively difficult to reduce electron-rich enamine int-2 to the undesired cyclic amine A ″. Fig. 1: Diastereoselective construction of functional polycyclic N-heterocycles by hydride transfer-initiated intermolecular annulation of the azaarenes. a The formation of N-alkyl enamine int-2 . b ruthenium-catalyzed dearomative annulation reaction of azaarenium salts A with aniline derivatives B and paraformaldehyde. c Selected drugs and bioactive molecules. Full size image Based on the above idea, we here report a dearomative annulation reaction of azaarenium salts A with aniline derivatives B and paraformaldehyde (Fig. 1b ) under ruthenium(II) reductive catalysis, which offers a general way for diastereoselective construction of fused syn -N-heterocycles P featuring promising structural motifs of teterahydroquinoline and hexahydro-1,6-naphthyridine that are frequently found in natural alkaloids [43] , [44] and biomedical molecules [45] , [46] , [47] , as exemplified by the leading anesthesia drug taripiprazole 1 , active composition 2 used for treating EP1 receptor-mediated diseases [45] , PXR agonist 3 [46] , and anticancer agents 4 (Fig. 1c ) [47] . Investigation of reaction conditions We commenced our studies by performing the reaction of N-benzyl quinolinium bromide A1 , N-ethylaniline B1 , paraformaldehyde, and base in MeOH at 65 °C for 18 h by employing [RuCl 2 ( p -cymene)] 2 as the catalyst. 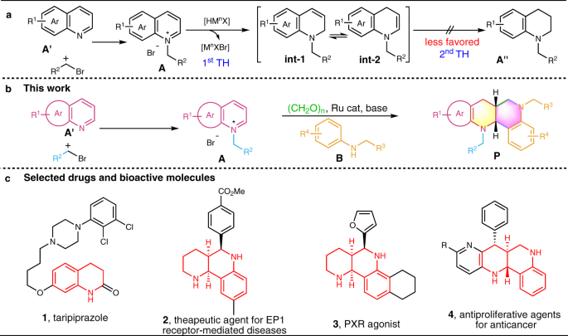Fig. 1: Diastereoselective construction of functional polycyclic N-heterocycles by hydride transfer-initiated intermolecular annulation of the azaarenes. aThe formation of N-alkyl enamineint-2.bruthenium-catalyzed dearomative annulation reaction of azaarenium salts A with aniline derivatives B and paraformaldehyde.cSelected drugs and bioactive molecules. Among various bases and acids tested, Mg(OMe) 2 exhibited the best chemo-selectivity since there is no formation of by-product N-benzyl tetrahydroquinoline A1″ (Table 1 , entries 1, 4 and Supplementary Table 1 in the Supplementary Information (SI) ). The absence of catalyst or base failed to yield product P1 (entries 5, 6), showing that both of them are indispensable for the product formation. Then, we screened several other metal catalysts applied frequently in hydrogen transfer reactions (see Supplementary Table 1 in SI). The results showed that Ir(I) or Ir(III) catalysts were also applicable, but the base metal catalysts (Co, Fe, Mn, and Ni) were totally ineffective for the transformation (entries 7, 8 and Supplementary Table 1 ). Here, we chose the cost-effective [Ru( p -cymene)Cl 2 ] 2 as the preferred catalyst to further evaluate the solvents and temperatures, it showed that methanol and 55 °C were more preferable (entries 9, 10). Decrease of the base or (CH 2 O) n amount diminished the product yields (entries 11, 12). Thus, the optimal yield of product P1 was obtained when the reaction in methanol was performed at 55 °C for 18 h by using the combination of [Ru( p -cymene)Cl 2 ] 2 and Mg(OMe) 2 (entry 10). Interestingly, the use of Mg(OMe) 2 base always resulted in excellent selectivity in affording product P1 (entries 3, and 7, 12). Table 1 The optimization of reaction conditions a . Full size table Substrate scope With the availability of the optimal reaction conditions (Table 1 , entry 10), we then assessed the substrate scope of the newly developed synthetic protocol. As shown in Fig. 2 , various quinolinium salts A ( A1 –A21 , see Supplementary Fig. 1 in SI for their structures) in combination with N-ethylaniline B1 and paraformaldehyde were evaluated. Gratifyingly, all the reactions underwent smooth reductive annulation and furnished the desired fused N-heterocycles in reasonable to excellent isolated yields with excellent syn -diastereoselectivity ( P1– P21 , d.r. > 20:1). The structure of compound P1 was confirmed by X-ray crystallography diffraction and NOESY spectrum (Supplementary Fig. 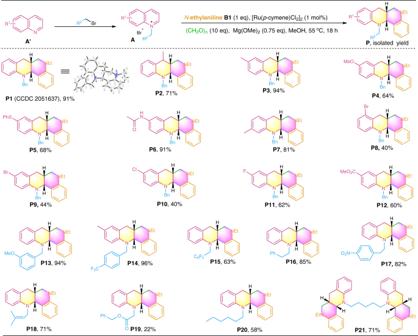Fig. 2: Diastereoselective construction of fused N-heterocyclesP1−P21by variation of quinolines. Reactions were conducted on a 0.2 mmol scale under the standard conditions. Isolated yields are reported. 3 – 5 and Supplementary Table 2 in SI). The application of 1,5-dibromopentane for di N-alkylation generated the intramolecular alkyl-linked product P21 in a good yield. Noteworthy, a variety of functionalities (e.g., −Me, −OMe, −SPh, amido, −F, −Cl, −Br, ester, −CF 3 , −NO 2 , alkenyl, and alkyl) on the quinolinium salts were well tolerated, and their electronic properties affected the product formation to some extent. Interestingly, no reduction of the nitro and alkenyl groups was observed ( P17 and P18 ), and the halo-substrates also did not undergo hydrodehalogenation, indicating that the reaction proceeds in a chemoselective manner. In general, quinolines bearing an electron-donating group ( P2– P7 , and P13– P14 ) afforded relatively higher product yields than those having an electron-withdrawing group ( P8 –P10 , and P12 ), presumably because the electron-rich quinolinium salts can result in more reactive enamine intermediates that are beneficial to the electrophilic coupling process (Fig. 1a ). The retention of these functionalities offers the potential for post-functionalization of the obtained products. Fig. 2: Diastereoselective construction of fused N-heterocycles P1 − P21 by variation of quinolines. Reactions were conducted on a 0.2 mmol scale under the standard conditions. Isolated yields are reported. Full size image Next, we turned our attention to the synthesis of structurally diversified products by variation of both azaarenes A′ and anilines B . First, a series of N-alkyl anilines ( B2 –B18 , see Supplementary Fig. 2 in SI for their structures) in combination with quinolinium salt A1 were tested. As illustrated in Fig. 3 , all the reactions efficiently afforded the desired product in moderate to excellent isolated yields with exclusive syn -selectivity ( P22 –P36 , d.r. > 20:1). The electronic properties of the substituents on the benzene ring of the anilines significantly affected the product formation. Especially, anilines containing electron-donating groups ( P2 2–P23 , P27 and P35 ) gave much higher yields than those with electron-withdrawing groups ( P2 4–P25 ). This observation is attributed to electron-rich anilines favoring the electrophilic coupling process during the formation of the products. In addition to N-alkyl anilines, diarylamine B13 also served as an effective coupling partner, affording the N-aryl product P33 in a moderate yield. As expected, primary anilines were not applicable for the transformation, as they easily reacted with formaldehyde to form aminals. Interestingly, tetrahydroquinolines ( B14 and B15 ) and 2,3,4,5-tetrahydro-1H-benzo[b]azepine ( B16 ), two specific aniline derivatives, also underwent efficient multicomponent annulation to afford the polycyclic products ( P34– P35 , P38 and P41 ). In addition to quinolines, other azaarenes, such as 1,8-naphthyridines ( A22 –A25 ), thieno[3,2-b]pyridine A26 , 1,7-phenanthroline A27 , 1,10-phenanthroline A28 , and 5-substituted isoquinolines ( A29 and A30 ) were also amenable to the transformation, delivering the desired products in an efficient manner ( P37– P49 , d.r. 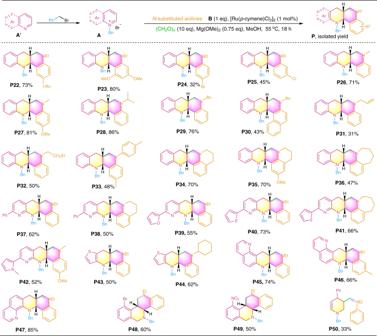Fig. 3: Diastereoselective access to fused N-heterocyclesP22–P50by variation of both azaarenes and anilines. Reactions were conducted on a 0.2 mmol scale under the standard conditions. Isolated yields are reported. > 20:1), these examples demonstrate the capability of the developed chemistry in the functionalization of pyridine-containing azaarenes including the N-bidentate ligands ( P37– P42 , P47 ). Unfortunately, more challenging pyridine derivative failed to yield the desired product, only β -aminoalkyl product ( P50 ) was obtained. Fig. 3: Diastereoselective access to fused N-heterocycles P22 – P50 by variation of both azaarenes and anilines. Reactions were conducted on a 0.2 mmol scale under the standard conditions. Isolated yields are reported. Full size image Noteworthy, 5-substituted isoquinolines afforded the desired annulation products (Fig. 3 , P48 and P49 ), whereas 5-nonsubstituted isoquinolines generated products P by installing an additional methyl group at the β -site of the N-heteroaryl reactants, and all the products are produced with exclusive syn -diastereoselectivity (d.r. > 20:1, Supplementary Fig. 6 ). As shown in Fig. 4 , N-benzyl isoquinolinium salts were firstly employed to couple with paraformaldehyde and N-ethylaniline B1 . All the reactions gave rise to the desired annulation products in moderate to excellent yields upon isolation ( P51– P63 ). Then, the transformation of secondary anilines including the N-alkyl and N-aryl ones was evaluated. Gratifyingly, all these anilines smoothly coupled with N-benzyl quinolium salt A1 and paraformaldehyde, delivering the annulation products in reasonable to high yields ( P64– P76 ). Similar to the results described in Figs. 2 and 3 , various functionalities on both isoquinolium salts and anilines are well tolerated (−Bn, −Et, −Me, −F, −Cl, −Br, boronic ester, −SO 2 Me, − n -hexyl, −OMe, −CF 3 , −CO 2 Me, alkenyl, cyclohexyl, and i -propyl). The substituents on the aryl ring of the isoquinoline salts have little influence on the product formation, whereas the substituents of the anilines significantly affected the product yields. Generally, aniline bearing an electron-donating group afforded higher yields (e.g., P64– P66 and P70– P73 ) than those of anilines with an electron-withdrawing group (e.g., P67 –P69 and P74 ), suggesting that the reaction involves an electrophilic coupling process. Benzocyclic amines (1,2,3,4-tetrahydroquinoxaline, 1,2,3,4-tetrahydroquinoline, and 2,3,4,5-tetrahydro-1H-benzo[b]azepine) and N1-isopropyl-N4-phenylbenzene-1,4-diamine also served as effective coupling partners, affording the polycyclic products in moderate to high yields ( P77 –P80 ). These examples show the practicality of the developed chemistry in the construction of structurally complex polycyclic N-heterocycles. Fig. 4: Diastereoselective access to fused N-heterocycles P51 – P80 by employing various isoquinolinium salts. Reactions were conducted on a 0.2 mmol scale under the standard conditions. Isolated yields are reported. Full size image Synthetic applications Further, we explored the synthetic applications of the developed chemistry. As shown in Fig. 5a , 6-ester quinolinium salts, arising from initial esterification of 6-carboxylic quinoline and subsequent pretreatment with benzyl bromide, efficiently reacted with aniline B1 and paraformaldehyde to afford products P81 and P82 (d.r. > 20:1), which are the analogs of analgesic [48] and the agents used for antioxidation and antiproliferation [49] , respectively. Through successive amidation and formation of N-benzyl heteroarenium salt, 6-amino quinoline was efficiently transformed in combination with aniline B1 into camphanic amide P83 (d.r. > 20:1, Fig. 5b ), an agent capable of stereoisomeric separation [50] . Further, the gram-scale synthesis of product P51 (d.r. > 20:1) was successfully achieved by scaling up the reactants to 10 mmol, which still gave a desirable yield (Fig. 5c ). Interestingly, representative compounds P29 and P51 underwent efficient debenzylation to afford N-unmasked products P84 (d.r. > 20:1) and P85 (d.r. > 20:1) in the presence of a Pd/HCOONH 4 system in methanol (Fig. 5d ), which demonstrates the practicality of the developed chemistry in further preparation of fused heterocycles containing a useful −NH motif. Fig. 5: Synthetic applications of the developed chemistry. a , b Structural modification of biomedical molecules. c Gram-scale synthesis. d Debenzylation of P29 and P51 . Full size image Mechanistic investigations To gain mechanistic insights into the reaction, we conducted several control experiments (Fig. 6 ). First, the model reaction was interrupted after 6 hours to analyze the product system. Except for the formation of product P1 in 23% yield, a dihydroquinoline int-1 was isolated in 5% yield (Fig. 6a ). Subjection of compound int-1 (Fig. 6a and Supplementary Fig. 8 ) with aniline B1 under the standard conditions resulted in product P1 in high isolated yield (Fig. 6b ), showing that int-1 is a key reaction intermediate. However, removal of Ru-catalyst from the standard conditions failed to produce P1 and the α-arylated product P1′ (Fig. 6c ), revealing that the reaction initiates with Ru-catalyzed hydrogen transfer, instead of nucleophilic arylation of substrate A1 with aniline B1 . Further, the model reaction using deuterated methanol solvent yielded product P1 without any D-incorporation (Fig. 6d ). In sharp contrast, the same reaction by replacing paraformaldehyde with the fully deuterated one gave product P1- d n with 35% and 28% D-ratios at the α and γ -sites and more than 99% D-ratio at the newly formed aminomethyl group (Fig. 6e and Supplementary Fig. 10 ). These two crucial experiments show that the formaldehyde serves as both the source of the reductant and C1-building block for the formation of the newly formed β -methylene group, and the initial reduction of A1 to give either int-1 or int-2 is reversible (Fig. 1a ). In parallel, we conducted the control experiments in terms of the generation of product P51 (Supplementary Fig. 7 in SI). The results also support that dihydroquinoline int-6 (Supplementary Fig. 7b ) and β -methyl dihydroquinoline int-9 (Supplementary Fig 9 ) are the reaction intermediates, and formaldehyde serves as the reductant source and C1-building block in the construction of the product (Supplementary Fig. 7d , e and Supplementary Fig. 11 ). Fig. 6: Control experiments for mechanistic studies. a Intermediate Detection. b Intermediate verification. c Ruling out possible reaction step. d , e Deuterium-labeling experiments to verify hydrogen donor and C1 source. Full size image Based on the above findings, the plausible pathways toward the formation products P1 and P51 are depicted in Fig. 7 . Initially, the metal hydride species [Ru II HX] is generated via Mg(OMe) 2 addition to formaldehyde ( E1 ) followed by transmetallation ( E2 ) with [Ru II X 2 ] and β -hydride elimination and release of formate ester (detected by GC-MS analysis, Supplementary Fig. 12 ). Then, the hydride transfer from [Ru II HX] to quinolinium salt A1 forms dihydroquinoline int-1 and its enamine tautomer int-2 along with regeneration of the catalyst precursor [Ru II X 2 ]. Meanwhile, the condensation between aniline B1 and formaldehyde affords iminium B1′ . Then, the β -nucleophilic addition of int-2 to B1′ gives the β -aminoalkyl iminium int-3 . Further, the electron-rich benzene ring of int-3 attacks the iminium motif from both the same ( int-3b ) and opposite ( int-3a ) sides of the H-atom at the β -site. In comparison, the form of int-3a (opposite side) is more favorable due to the less steric hindrance, thus affording product P1 with syn -selectivity after deprotonation of the coupling adduct int-4 (path a of Fig. 7b , namely electrophilic aryl C–H aminoalkylation). Alternatively, the [4 + 2] cycloaddition of int-2 and B1′ via endo or exo π-π stacking also rationalizes the formation of int-4 and product P1 (path b of Fig. 7b , via int-5 and int −4 ). Similarly, the generation of product P51 from isoquinoline is shown in Fig. 6c . The hydride transfer from [Ru II HX] to isoquinolinium salt A32 initially forms enamine int-6 (Supplementary Fig. 7a , b and Fig. 8). Then, the β -capture of formaldehyde by int-6 followed by based-facilitated dehydration of int-7 and hydride transfer to alkenyl iminium salt int-8 forms β -methyl enamine int-9 (Supplementary Fig. 7a and Fig. 9 ). Subsequently, the β -capture of B1′ by int-9 followed by intramolecular attack of the electron-rich phenyl ring to the iminium motif of int-10 from the sterically less hindered back side of the methyl group, or the [4 + 2] cycloaddition of int-9 and B1′ via π-π stacking gives intermediate int-11 . Finally, the deprotonation of int-11 generates product P51 with syn -diastereoselectivity (Fig. 7c ). Fig. 7: Plausible reaction mechanism. a The production of metal hydride species. b Possible pathways for the formation product P1 . c Possible pathway for the formation product P51 . Full size image Fig. 8: DFT studies (free energies in kcal mol −1 ). a Potential energy surfaces for the process from int-2 to P1 . b Potential energy surfaces for the process from int-6 to P51 . Full size image To better reveal the selective formation of products P1 and P51 , computational study was performed using the density functional theory and the relevant data was listed in the Supplementary Dataset file. First, the participation of Mg(OMe) 2 , MeOK, and t -BuOK as the bases in the generation of [Ru II HCl] was calculated. The energy for the transmetallation step with Mg(OMe) 2 ( int-22 → int-23 , Δ G = 10.1 kcal mol −1 in supplementary Fig. 13 ) is significantly higher than the other two bases ( int-26 → int-27 , Δ G = −3.6 kcal mol −1 for t -BuOK in supplementary Fig. 14 ; int-30 → int-23 , Δ G = −0.6 kcal mol −1 for MeOK in supplementary Fig. 15 ). The results reveal that the Mg 2+ ion can better stabilize adduct E1 (Fig. 7a ) and make the dissociation of -MgOMe as well as the transmetallation process more difficult, thus resulting in a slow forming rate of [Ru II HCl]. Correspondingly, a slow generation of enamine int-2 via hydride transfer from [Ru II HCl] to azaarenium salt A1 is beneficial to the capture of int-2 by B1′ , and effectively suppresses the formation of undesired N-benzyl tetrahydroquinoline A1″ (Table 1 ). Next, the free energy profile for the conversion of int-2 and B1′ to P1 is depicted in Fig. 8a and supplementary Fig. 16 . The formation of int-3a and int-3b via β -nucleophilic addition of int-2 to B1′ has the energy barriers of 14.0 kcal mol −1 ( TS4 ) and 14.5 kcal mol −1 ( TS4′ ), respectively, representing endothermic processes (Δ G = 6.3 kcal·mol −1 and Δ G = 5.6 kcal·mol −1 ). The only difference between int-3a and int-3b is the dihedral of C2-C3-N2-C4 ( int-3a , −76.0° vs int-3b , 106.9°), and the conversion of int-3a to int-3b is rather easy with only an energy barrier of 8.7 kcal·mol −1 . However, int-3b is not a favorable intermediate, as it has high stereoscopic hindrance of the N-ethyl group and pyridyl β -H as well as the long distance (~5.7 Å) between the pyridyl α -carbon (C1) and aniline ortho -carbon (C5). Therefore, int-3a becomes a favorable intermediate, and the attack of electron-rich aryl group to electron-deficient iminium motif generates int-4 by intramolecular C1–C5 bond formation with an energy barrier of 15.5 kcal mol −1 ( TS6 ). Finally, the formation of product P1 , via deprotonative aromatization of int-4 , is a thermodynamically favorable process from the energetic point of view (Δ G = −54.1 kcal mol −1 ). In terms of the [4 + 2] cycloaddition of B1′ and int-2 , the manner of endo π-π stacking encountered commonly in the Diels-Alder reactions has a significant energy barrier of 39.0 kcal mol −1 ( TS7 ). So, this pathway is disfavored. 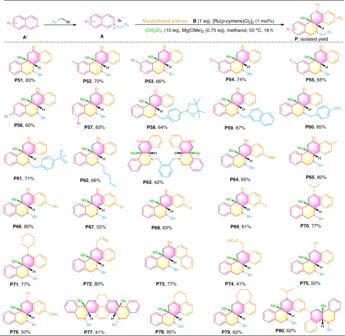Fig. 4: Diastereoselective access to fused N-heterocyclesP51–P80by employing various isoquinolinium salts. Reactions were conducted on a 0.2 mmol scale under the standard conditions. Isolated yields are reported. Meanwhile, the calculation results show that the manner of exo π-π stacking is also difficult to take place due to the higher steric hindrance and long interaction distance. Based on the computational studies, path a shown in Fig. 7b is believed to be a favorable way in generating product P1 . Further, the calculation results for the generation of product P51 are depicted in Fig. 8b and supplementary Fig. 17 . The formation of requisite intermediate int-9 involves four main steps: (i) the β -addition of int-6 to HCHO ( int-6 → int-6′ ), (ii) proton transfer from the methanol ( int-6′ → int-7 ), (iii) Mg(OMe) 2 -induced proton abstraction and dissociation of OH - ( int-7 → int-7′ → int-8 ), and (iv) hydride transfer ( int-8 → int-9 ). Noteworthy, from step (i) to (iii), the formation of int-8 clearly proceeds under the assistance of Mg 2+ , and these steps can easily take place with a maximum energy barrier of 8.8 kcal·mol −1 ( TS8 ). 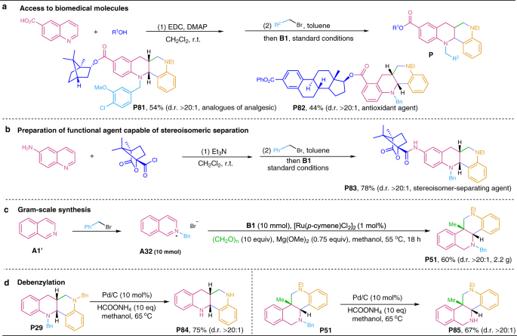Fig. 5: Synthetic applications of the developed chemistry. a,bStructural modification of biomedical molecules.cGram-scale synthesis.dDebenzylation ofP29andP51. Next, the formation of int-9 by hydride transfer from [Ru II HCl] complex to int-8 proceeds with an energy barrier of 11.6 kcal·mol −1 ( TS11 ), which is exothermic process (ΔG = − 6.1 kcal mol −1 ). Once int-9 is formed, the generation product P51 proceeds with a similar way of Fig. 8a : β -addition of int-9 to B1′ , intramolecular cyclization via C1–C5 bond formation, and based-promoted deprotonation of int-11 to yield product P51 . The calculation results show that the processes from int-9 to P51 have a slightly higher barrier than that of generating P1 in Fig. 8a (Δ G ≠ = 17.5 kcal mol −1 for TS13 vs Δ G ≠ = 15.5 kcal mol −1 for TS6 ). In summary, by a strategy incorporating a tandem coupling sequence into the reduction of azaarenium salts, we have developed a intermolecular syn -diastereoselective annulation reaction by reductive ruthenium(II) catalysis. A variety of azaarenes were efficiently transformed in combination with a large variety of aniline derivatives into fused N-heterocycles by employing paraformaldehyde as both a crucial agent to generate active ruthenium(II)-hydride species and a C1-building block, proceeding with readily available feedstocks, excellent selectivity, mild conditions, and broad substrate and functional group compatibility. The present work has established a practical platform for the transformation of ubiquitously distributed but weakly reactive azaarenes into functional organic frameworks that are difficult accessible with the existing approaches, and further discovery of bioactive and drug-relevant molecules due to the promising potentials of the obtained compounds featuring the teterahydroquinolyl and hexahydro-1,6-naphthyridyl motifs. Mechanistic studies reveal that the products are formed via hydride transfer-initiated β -aminomethylation and α -arylation of the azaarenium salts, and the use of Mg(OMe) 2 as a base plays a critical role in determining the reaction chemo-selectivity by lowering the hydrogen transfer rate. The work presented fills an important gap in the capabilities of utilizing azaarenes as the synthons to access fused N-heterocycles, and opens a door to further develop valuable reductive functionalization of inert unsaturated systems by taking profit of formaldehyde-endowed two functions. Typical procedure I for the synthesis of product P1 Under N 2 atmosphere, [Ru( p -cymene)Cl 2 ] 2 (1 mol %), 1-benzylquinolin-1-ium bromide A1 (0.2 mmol), N-ethylaniline B1 (0.2 mmol), Mg(OMe) 2 (0.75 eq, 12.9 mg), (CH 2 O) n (10.0 eq, 60 mg) and methanol (1 mL) were introduced in a Schlenk tube, successively. Then the Schlenk tube was closed and the resulting mixture was stirred at 55 °C for 18 h. After cooling down to room temperature, the mixture was extracted with ethyl acetate, washed with 5% Na 2 CO 3 solution, dried with anhydrous sodium sulfate, and then concentrated by removing the solvent under vacuum. Finally, the residue was purified by preparative TLC on silica to give 12-benzyl-5-ethyl-5,6,6a,7,12,12a-hexahydrodibenzo[ b,h ][1,6]naphthyridine P1 . See Supplementary methods for the structure and synthesis methods of the employed substrates, intermediates and utility. 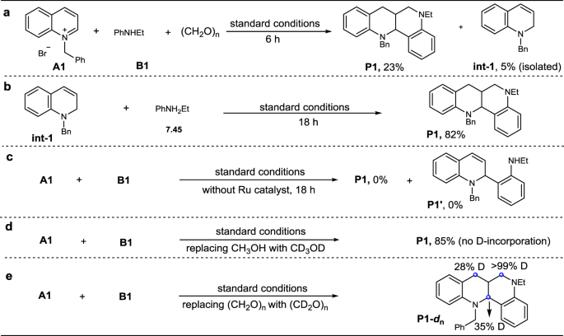Fig. 6: Control experiments for mechanistic studies. aIntermediate Detection.bIntermediate verification.cRuling out possible reaction step.d,eDeuterium-labeling experiments to verify hydrogen donor and C1 source. The analytical data and NMR spectra of all obtained compounds ( P1 – P85 , int-1 and int-6 ) are presented within Supplementary Information . See Supplementary Figs. 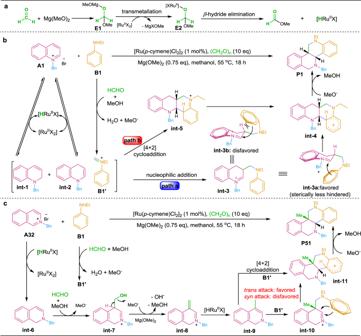Fig. 7: Plausible reaction mechanism. aThe production of metal hydride species.bPossible pathways for the formation productP1.cPossible pathway for the formation productP51. 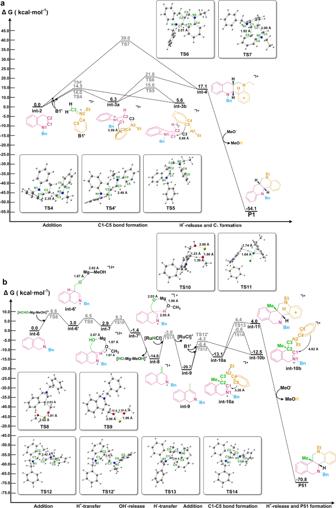Fig. 8: DFT studies (free energies in kcal mol−1). aPotential energy surfaces for the process fromint-2toP1.bPotential energy surfaces for the process fromint-6toP51. 18 – 197 for NMR spectroscopic data of all compounds.